A biosensor to monitor dynamic regulation and function of tumour suppressor PTEN in living cells Tumour suppressor PTEN is a phosphatase that negatively regulates the PI3K/AKT pathway. The ability to directly monitor PTEN conformation and function in a rapid, sensitive manner is a key step towards developing anti-cancer drugs aimed at enhancing or restoring PTEN-dependent pathways. Here we developed an intramolecular bioluminescence resonance energy transfer (BRET)-based biosensor, capable of detecting signal-dependent PTEN conformational changes in live cells. The biosensor retains intrinsic properties of PTEN, enabling structure–function and kinetic analyses. BRET shifts, indicating conformational change, were detected following mutations that disrupt intramolecular PTEN interactions, promoting plasma membrane targeting and also following physiological PTEN activation. Using the biosensor as a reporter, we uncovered PTEN activation by several G protein-coupled receptors, previously unknown as PTEN regulators. Trastuzumab, used to treat ERBB2-overexpressing breast cancers also elicited activation-associated PTEN conformational rearrangement. We propose the biosensor can be used to identify pathways regulating PTEN or molecules that enhance its anti-tumour activity. Tumour suppressor PTEN (phosphatase and tensin homologue deleted on chromosome 10) is a lipid phosphatase that dephosphorylates phosphatidyl (3,4,5) trisphosphate (PIP3) and thus inhibits phosphoinositide 3-kinase (PI3K)/AKT signalling. By opposing the PI3K/AKT pathway, PTEN regulates cell proliferation, survival and migration. Loss of PTEN function occurs in a broad range of human cancers, and it is often mutated in inherited cancer-predisposition syndromes such as Cowden disease [1] , [2] , [3] . In cultured cells, deletion of the PTEN gene, or reduction of PTEN levels using RNA interference, leads to increased PIP3-dependent AKT activation. In vivo studies have also addressed the importance of PTEN in the development of cancer. Whereas homozygous deletion of Pten leads to early embryonic death, Pten +/− mice develop various cancers and also a lethal lymphoproliferative disease [4] . Furthermore, studies employing genetic manipulation of Pten to produce a series of mice carrying different combinations of wild-type, null and hypomorphic alleles, have demonstrated that subtle reductions in Pten levels are sufficient to promote cancer susceptibility [5] , [6] . Regulation of PTEN levels, localization and activity are subject to tight control. PTEN expression is controlled by numerous transcription factors (for example, p53, Egr-1 and CBF-1) and post-transcriptionally via oncogenic microRNAs that target PTEN mRNA [1] , [2] . Recently, it was shown that both mRNAs of the PTEN pseudogene, PTENP1 , and competing endogenous RNAs could serve as decoys for PTEN mRNA-targeting microRNAs, inhibiting their effects on PTEN expression [7] , [8] . PTEN is also regulated through protein–protein interactions, the association of scaffolding proteins such as MAGI-1 and -2, NHERF and β-arrestins (β-arrs) altering its function and/or subcellular localization [9] , [10] , [11] , [12] . Finally, PTEN catalytic activity is regulated post-translationally by phosphorylation, acetylation, SUMOylation and ubiquitination [2] , [13] . Phosphorylation is the best-characterized post-translational mechanism of PTEN regulation. The PTEN protein is composed of a short amino-terminal PIP2-binding motif, a catalytic domain, C2 domain and a regulatory carboxy-terminal tail [1] , [14] . A cluster of serine and threonine residues (Ser380, Thr382, Thr383 and Ser385) in the regulatory C-terminal tail of PTEN is constitutively phosphorylated by casein kinase 2 (CK2). This results in a stable ‘closed’ form that has reduced lipid phosphatase activity, decreased plasma membrane targeting and increased conformational compaction [15] , [16] , [17] , [18] , [19] . Intramolecular interaction of the phosphorylated C-terminal tail with basic residues within the N-terminal PIP2-binding motif, the catalytic and C2 domains, maintains PTEN in its ‘closed’ form [20] , [21] . Mutation of the C-terminal tail phosphorylation cluster disrupts the intramolecular interaction and promotes an ‘open’ form of PTEN with increased catalytic activity and plasma membrane targeting. These findings have led to an elegant model whereby a phosphorylation-regulated switch controls the transition of PTEN from a ‘closed’ cytoplasmic inactive state and an ‘open’ active state that is localized to the plasma membrane [17] , [19] , [21] . PTEN is also phosphorylated in its C2 domain by ROCK, the downstream effector of RhoA, resulting in increased PTEN catalytic activity [22] . Finally, PTEN function can be inhibited by phosphorylation on tyrosine residues by Src family kinases [23] , [24] . Phosphorylation of tyrosine residues, in the C2 domain, are thought to inhibit binding of PTEN to cellular membranes, thus leading to increased PI3K/AKT signalling [23] , [24] . Downregulation of PTEN activity in human cancers can occur via post-translational modification, in the absence of any PTEN gene alteration. For example, in T-cell acute lymphoblastic leukemia (T-ALL), PTEN is mostly inactivated by phosphorylation and oxidation, resulting in hyperactivation of the PI3K/AKT pathway [25] . Pharmacological manipulation of the post-translational mechanisms inactivating PTEN restored PTEN activity and inhibited PI3K/AKT signalling in T-ALL cells [25] . The ability to directly monitor PTEN, in a rapid and sensitive manner, is a key issue to speed the development of anti-cancer drugs aimed at enhancing or restoring PTEN-dependent cellular pathways. Indeed, direct measurement of PTEN activity can currently only be assessed by enzymatic end point assays in cell lysates. We have therefore developed an intramolecular bioluminescence resonance energy transfer (BRET)-based biosensor that can be used in intact live cells to detect conformational changes of PTEN. Using the biosensor, we were able to detect conformational rearrangement of PTEN induced by (i) targeted mutation of phosphorylation sites affecting key intramolecular interactions as well as cancer-associated mutations ablating major mono-ubiquitination sites, (ii) modulation of signalling pathways that impact PTEN function, including novel G protein-coupled receptor (GPCR)-mediated regulation and (iii) the therapeutic agent trastuzumab, used in the treatment of ERBB2-overexpressing breast cancers. Establishment and validation of the Rluc-PTEN-YFP biosensor Biosensors based on intramolecular resonance energy transfer (RET) detect molecular proximity between donor and acceptor molecules at the nanometre scale [26] . Changes in intramolecular RET, depending on the relative orientation of the donor and acceptor proteins in the fusion, permit the monitoring of conformational changes in the ‘test’ protein sandwiched between the donor/acceptor couple [26] , [27] . To determine whether changes in PTEN conformation can be followed in live cells, we set up an intramolecular BRET-based biosensor, comprising the energy donor, Rluc, fused to the amino terminus of PTEN and the energy acceptor, yellow fluorescent protein (YFP), fused to the carboxy terminus of PTEN ( Fig. 1a ). Importantly, the lipid phosphatase catalytic activity of PTEN in the Rluc-PTEN-YFP biosensor remained intact, as shown by an in vitro assay that measures free phosphate released from PIP3 ( Fig. 1b ). PTEN-null prostate cancer PC-3 cells transfected with Rluc-PTEN-YFP were lysed and catalytic activity of immunoprecipitated PTEN measured. Lipid phosphatase activity of the PTEN biosensor was assessed by measurement of released phosphate from PIP3, YFP-transfected cells serving as control ( Fig. 1b ). As the lipid phosphatase activity of PTEN antagonizes the PI3K/AKT signalling pathway, through conversion of PIP3 to PIP2, we next tested the functional activity of the biosensor using AKT activation as readout. Expression of Rluc-PTEN-YFP in PC-3 cells resulted in decreased AKT activation as indicated by reduced pAKT levels compared with empty vector-transfected cells ( Fig. 1c ). This was comparable to a Myc-tagged form of PTEN and PTEN-YFP expressed at similar levels ( Fig. 1c ). In addition, Rluc-PTEN-YFP displayed a similar cellular distribution to PTEN-YFP when imaged in live HEK cells, being found mainly in the cytoplasm, but also in the nucleus ( Fig. 1d ), consistent with previous reports [21] . Finally, Rluc-PTEN-YFP retained the capacity to interact with protein partners as shown by the co-immunoprecipitation of the molecular scaffold β-arr2 (ref. 11 ) with the biosensor ( Fig. 1e ). Taken together, these results indicate that PTEN maintains its functional repertoire within the Rluc-PTEN-YFP biosensor. 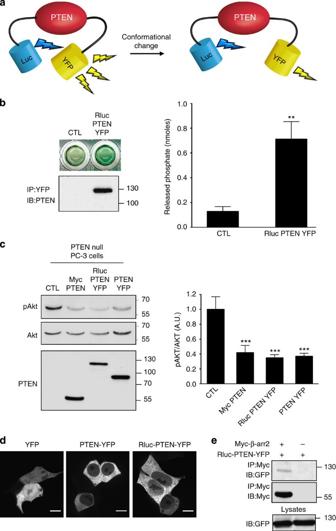Figure 1: The Rluc-PTEN-YFP biosensor retains PTEN functionality. (a) Schematic representation of Rluc-PTEN-YFP biosensor. PTEN is sandwiched between Rluc (Luc in diagram) and YFP. This diagram illustrates how conformational changes may induce variations in BRET measurements, although the real orientations of donor and acceptor proteins are not known. (b) PTEN immunoprecipitates from PC-3 cells expressing YFP or Rluc-PTEN-YFP were analysed for the capacity to dephosphorylate water-soluble diC8-PIP3 (100 μM). Data shown represent mean±s.e.m. of three independent experiments. **P<0.01,t-test. (c) Levels of activated Akt (pAkt Ser 473) measured in PC-3 cells recomplemented with Myc-PTEN, Rluc-PTEN-YFP or PTEN-YFP. Histogram represents quantification of relative pAkt levels for four independent experiments. A.U., arbitrary units. ***P<0.001, analysis of variance with Bonferronipost hoctest. (d) Subcellular distribution of YFP, PTEN-YFP and Rluc-PTEN-YFP. HEK cells were transfected with the indicated plasmids and live cells were imaged. Scale bar, 10 μm. (e) Co-immunoprecipitation of Rluc-PTEN-YFP with Myc-β-arr2 from transfected HEK293 cells. Myc-β-arr2 was immunoprecipitated using anti-myc antibodies and associated Rluc-PTEN-YFP was revealed with an anti-green fluorescent protein antibody. Figure 1: The Rluc-PTEN-YFP biosensor retains PTEN functionality. ( a ) Schematic representation of Rluc-PTEN-YFP biosensor. PTEN is sandwiched between Rluc (Luc in diagram) and YFP. This diagram illustrates how conformational changes may induce variations in BRET measurements, although the real orientations of donor and acceptor proteins are not known. ( b ) PTEN immunoprecipitates from PC-3 cells expressing YFP or Rluc-PTEN-YFP were analysed for the capacity to dephosphorylate water-soluble diC8-PIP3 (100 μM). Data shown represent mean±s.e.m. of three independent experiments. ** P <0.01, t -test. ( c ) Levels of activated Akt (pAkt Ser 473) measured in PC-3 cells recomplemented with Myc-PTEN, Rluc-PTEN-YFP or PTEN-YFP. Histogram represents quantification of relative pAkt levels for four independent experiments. A.U., arbitrary units. *** P <0.001, analysis of variance with Bonferroni post hoc test. ( d ) Subcellular distribution of YFP, PTEN-YFP and Rluc-PTEN-YFP. HEK cells were transfected with the indicated plasmids and live cells were imaged. Scale bar, 10 μm. ( e ) Co-immunoprecipitation of Rluc-PTEN-YFP with Myc-β-arr2 from transfected HEK293 cells. Myc-β-arr2 was immunoprecipitated using anti-myc antibodies and associated Rluc-PTEN-YFP was revealed with an anti-green fluorescent protein antibody. Full size image In HEK cells expressing Rluc-PTEN-YFP, addition of the membrane-permeable substrate for Rluc, coelenterazine h , elicited a strong basal BRET signal (~300 mBRET), indicating molecular proximity of the donor and acceptor in the biosensor ( Fig. 2a ). To eliminate the possibility that the signal detected could be due to intermolecular BRET between adjacent Rluc-PTEN-YFP molecules, we measured the BRET signal obtained with separate Rluc-PTEN and PTEN-YFP fusion proteins. Cells coexpressing Rluc-PTEN and PTEN-YFP at equivalent luminescence and fluorescence levels ( Supplementary Fig. 1a,b ) as those obtained with Rluc-PTEN-YFP gave a minimal basal BRET ( Fig. 2a ), indicating that the signal detected with Rluc-PTEN-YFP does indeed reflect intramolecular BRET. We next tested whether BRET could be detected in cells expressing ‘physiological’ levels of the PTEN biosensor. For this, we transfected PTEN-null PC-3 cells with Rluc-PTEN-YFP to levels approximating endogenous levels of PTEN in HEK cells, with over 30% of PC-3 cells transfected under these conditions ( Fig. 2b and Supplementary Fig. 1c ). Using this approach, we were able to detect a BRET signal ( Fig. 2a ), indicating that the biosensor can indeed be used at ‘physiological’ expression levels. As expected for the donor and acceptor being contained in the same molecule, the BRET signal remained stable with increasing Rluc values over >100-fold range ( Fig. 2c and d ), due to the constant acceptor to donor ratio [28] . 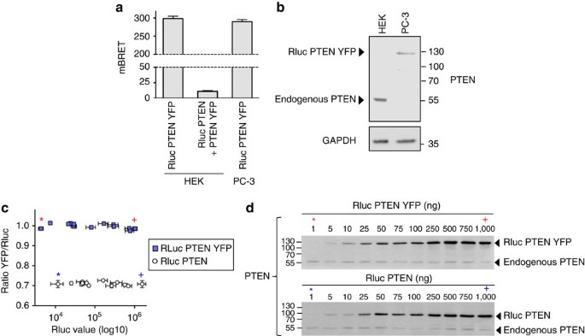Figure 2: Intramolecular BRET signals of Rluc-PTEN-YFP. (a) mBRET measurements in HEK293 cells transfected with Rluc-PTEN-YFP for intramolecular BRET, or cotransfected with Rluc-PTEN and PTEN-YFP for intermolecular BRET. PC-3 cells were transfected with Rluc-PTEN-YFP at levels comparable to endogenous PTEN in HEK cells as shown in western blotting (b). Data are mean±s.e.m. of four independent experiments. (c) BRET measurements for increasing concentrations of the indicated constructs. Data are mean±s.e.m. of four independent experiments. (d) Representative blots using an anti-PTEN antibody. Symbols (*) and (+) refer to their respective BRET measurements inc. BRET measurements in these experiments were performed on detached cells. Figure 2: Intramolecular BRET signals of Rluc-PTEN-YFP. ( a ) mBRET measurements in HEK293 cells transfected with Rluc-PTEN-YFP for intramolecular BRET, or cotransfected with Rluc-PTEN and PTEN-YFP for intermolecular BRET. PC-3 cells were transfected with Rluc-PTEN-YFP at levels comparable to endogenous PTEN in HEK cells as shown in western blotting ( b ). Data are mean±s.e.m. of four independent experiments. ( c ) BRET measurements for increasing concentrations of the indicated constructs. Data are mean±s.e.m. of four independent experiments. ( d ) Representative blots using an anti-PTEN antibody. Symbols (*) and (+) refer to their respective BRET measurements in c . BRET measurements in these experiments were performed on detached cells. Full size image Rluc-PTEN-YFP reports PTEN functional change in live cells Phosphorylation of PTEN in its C-terminal tail on residues Ser380, Thr382, Thr383 and Ser385 ( Fig. 3a ) favours the closed, predominantly cytoplasmic, form of PTEN [16] , [17] , [18] . Dephosphorylation of these residues promotes an open, active form of PTEN that is targeted to the plasma membrane. As reported previously [21] , the C-terminal tail of PTEN (PTEN-tail, amino acids 356–403) can be co-immunoprecipitated with a truncated form of PTEN lacking the C-terminal tail (PTEN-Δtail, amino acids 1–355; Supplementary Fig. 2a ). Mutation of the phosphorylation cluster to alanine residues (Ser380Ala, Thr382Ala, Thr383Ala and Ser385Ala) results in loss of binding between PTEN-Δtail and PTEN-tail ( Supplementary Fig. 2a ). Furthermore, whereas full-length PTEN does not associate with a coexpressed C-terminal tail, a full-length form of PTEN mutated in its phosphorylation cluster (PTEN-A4) is able to associate with the tail ( Supplementary Fig. 2b ). These data are consistent with the proposed model of a phosphorylation-dependent intramolecular interaction between amino acids 356–403 in the PTEN C-tail and residues contained within amino acids 1–355 of PTEN-Δtail. 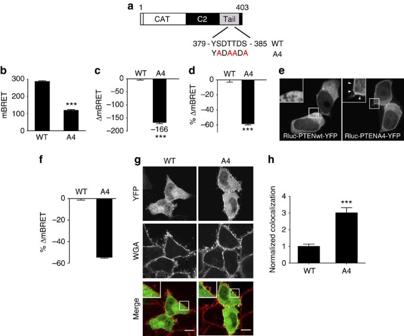Figure 3: Conformational change of PTEN monitored by BRET following mutation of key regulatory residues. (a) Schematic representation of PTEN showing the regulatory phosphorylation site residues in the C-terminal tail and the mutation introduced to create the PTEN-A4 mutant. Respective mBRET (b), ΔmBRET (c) and %ΔmBRET (d) values of Rluc-PTENwt-YFP and Rluc-PTEN(A4)-YFP. The graphs represent mean±s.e.m. of four independent experiments. ***P<0.001,t-test. (e) Localization of PTEN constructs in HEK cells. Cells were transfected with Rluc-PTENwt-YFP and Rluc-PTEN(A4)-YFP, and live cells were imaged. Insets show magnified regions of the boxed areas and demonstrate membrane targeting of PTEN-A4 (arrowheads). (f) % ΔmBRET of Rluc-PTEN(A4)-YFP versus Rluc-PTENwt-YFP in HeLa cells. Error bars are s.e.m. (g,h) Colocalization of Rluc-PTEN-YFP and Rluc-PTEN(A4)-YFP with fluorescent-wheat germ agglutinin (WGA) on non-permebilized HeLa cells. Insets show magnified regions of the boxed regions. Scale bars, 10 μm. Quantification mean±s.e.m. on 12 different cells was performed using the Image J colocalization plugin, ***P<0.001,t-test. BRET measurements in these experiments were performed on detached cells. Figure 3: Conformational change of PTEN monitored by BRET following mutation of key regulatory residues. ( a ) Schematic representation of PTEN showing the regulatory phosphorylation site residues in the C-terminal tail and the mutation introduced to create the PTEN-A4 mutant. Respective mBRET ( b ), ΔmBRET ( c ) and %ΔmBRET ( d ) values of Rluc-PTENwt-YFP and Rluc-PTEN(A4)-YFP. The graphs represent mean±s.e.m. of four independent experiments. *** P <0.001, t -test. ( e ) Localization of PTEN constructs in HEK cells. Cells were transfected with Rluc-PTENwt-YFP and Rluc-PTEN(A4)-YFP, and live cells were imaged. Insets show magnified regions of the boxed areas and demonstrate membrane targeting of PTEN-A4 (arrowheads). ( f ) % ΔmBRET of Rluc-PTEN(A4)-YFP versus Rluc-PTENwt-YFP in HeLa cells. Error bars are s.e.m. ( g , h ) Colocalization of Rluc-PTEN-YFP and Rluc-PTEN(A4)-YFP with fluorescent-wheat germ agglutinin (WGA) on non-permebilized HeLa cells. Insets show magnified regions of the boxed regions. Scale bars, 10 μm. Quantification mean±s.e.m. on 12 different cells was performed using the Image J colocalization plugin, *** P <0.001, t -test. BRET measurements in these experiments were performed on detached cells. Full size image To determine whether PTEN conformational changes can be monitored in live cells, we introduced Ser380Ala, Thr382Ala, Thr383Ala and Ser385Ala mutations in the biosensor (Rluc-PTEN(A4)-YFP) ( Fig. 3a ). Strikingly, mutation of all four phosphorylation residues within Rluc-PTEN-YFP produced a marked reduction in the BRET signal (>50%), compared with wild-type PTEN, indicating increased distance and or/altered orientation of Rluc and YFP relative to each other ( Fig. 3b–d ). This change is consistent with the ‘opening’ of the PTEN molecule on dephosphorylation of its C-terminal tail in live HEK cells. The change in BRET signal observed with Rluc-PTEN(A4)-YFP was associated with increased targeting to the plasma membrane in live HEK cells ( Fig. 3e ). A similar decrease in BRET with Rluc-PTEN(A4)-YFP was observed in HeLa cells ( Fig. 3f ). Again, this was associated with enhanced membrane targeting as assessed by increased colocalization of YFP signal with red fluorescent-labelled lectin, wheat germ agglutinin, on non-permeabilized cells ( Fig. 3g,h ). These data demonstrate that conformational change of PTEN can be monitored in live cells using the biosensor. Pathways controlling PTEN are detected by Rluc-PTEN-YFP We next examined whether signalling pathways known to regulate PTEN activity would induce BRET changes in cells expressing Rluc-PTEN-YFP. The serine-threonine kinase CK2 is involved in phosphorylation of the regulatory sites in the C terminus of PTEN. CK2 overexpression has been observed in several different types of cancer [25] , [29] , [30] , [31] . For example, in human T-ALL, CK2 is overexpressed, leading to phospho-dependent PTEN inactivation and subsequent hyperactivation of the PI3K/AKT pathway [25] . Pharmacological inhibition of CK2 restored PTEN activity and inhibited PI3K/AKT signalling in T-ALL cells [25] . We examined whether incubation of cells with the CK2 inhibitor, tetrabromobenzotriazole (TBB), could modulate the BRET signal of Rluc-PTEN-YFP ( Fig. 4a–c ). For this, we transfected PC-3 cells with the PTEN biosensor and incubated cells overnight with the CK2 inhibitor. Consistent with our results using the C-terminal mutants above, TBB elicited a significant decrease in BRET ( P <0.001, n =4, t -test), which parallelled a significant decrease ( P <0.05, n =4, t -test) in phosphorylation of Ser380/Thr382/Thr383 as assessed with a specific phospho-PTEN antibody against these sites ( Fig. 4a–c ). Cells incubated with TBB also displayed decreased pAKT levels ( Fig. 4d,e ) consistent with previous reports [25] . In a converse approach to CK2 inhibition, we next assessed the effect of co-expressed HA-tagged CK2 on the biosensor. Interestingly, HA-CK2 elicited a significant increase ( P <0.001) above baseline BRET of the biosensor ( Fig. 4f ) as opposed to the decrease observed with TBB. These results indicate that both positive and negative modification of signalling pathways that impact on PTEN function can be detected using the biosensor in live cells. 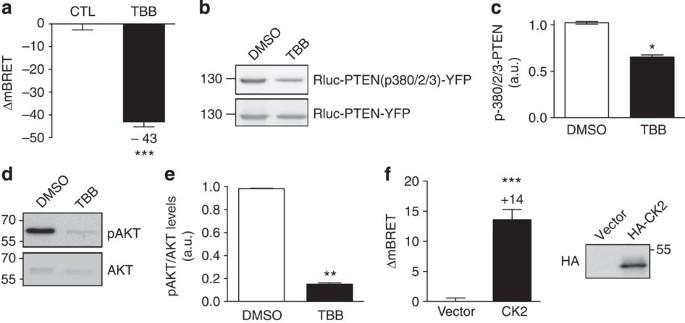Figure 4: Modulation of CK2 promotes conformational changes in PTEN. (a–c) Effect of overnight incubation with the CK2 inhibitor, TBB (50 μM), on BRET signal (a) and phosphorylation of the S380/T382/T383 cluster (b,c) in PC-3 cells transfected with Rluc-PTEN-YFP. The graphs represent mean±s.e.m. of four independent experiments. A.U., arbitrary units. ***P<0.001, *P<0.05,t-tests. (d,e) Effect of TBB incubation on pAKT levels in serum-starved PC-3 cells transfected with Rluc-PTEN-YFP. The graph represents mean±s.e.m. of four independent experiments. A.U., arbitrary units. **P<0.01,t-test. (f) Effect of overexpression of HA-CK2 on BRET of Rluc-PTEN-YFP in HEK cells. The graph represents mean±s.e.m. of four independent experiments. ***P<0.001,t-test. BRET measurements in these experiments were performed on detached cells. Figure 4: Modulation of CK2 promotes conformational changes in PTEN. ( a – c ) Effect of overnight incubation with the CK2 inhibitor, TBB (50 μM), on BRET signal ( a ) and phosphorylation of the S380/T382/T383 cluster ( b , c ) in PC-3 cells transfected with Rluc-PTEN-YFP. The graphs represent mean±s.e.m. of four independent experiments. A.U., arbitrary units. *** P <0.001, * P <0.05, t -tests. ( d , e ) Effect of TBB incubation on pAKT levels in serum-starved PC-3 cells transfected with Rluc-PTEN-YFP. The graph represents mean±s.e.m. of four independent experiments. A.U., arbitrary units. ** P <0.01, t -test. ( f ) Effect of overexpression of HA-CK2 on BRET of Rluc-PTEN-YFP in HEK cells. The graph represents mean±s.e.m. of four independent experiments. *** P <0.001, t -test. BRET measurements in these experiments were performed on detached cells. Full size image We next investigated the effect of the RhoA/ROCK pathway on Rluc-PTEN-YFP, as the small GTPase RhoA is known to stimulate PTEN activity via its downstream effector ROCK [11] , [22] , [32] . We coexpressed the PTEN biosensor with a constitutively active form of RhoA (RhoA-V14). RhoA-V14 produced a robust decrease in BRET compared with vector-transfected cells ( Fig. 5a ), indicating conformational change, and activation of the biosensor, as shown by in vitro phosphatase assay ( Fig. 5b ), as well as reduced pAKT levels in cells ( Fig. 5c ). We recently showed that β-arrs bind directly and activate PTEN lipid phosphatase activity and that this occurs downstream of RhoA/ROCK signalling [11] . We thus tested the effect of β-arr2 on PTEN conformation using the biosensor. Coexpression of Rluc-PTEN-YFP with β-arr2 induced both a reduction in BRET and increased lipid phosphatase activity ( Fig. 5d,e ). We also made use of β-arr2−/− mouse embryonic flibroblasts for effects on the biosensor. Compared with wild-type counterparts, β-arr2−/− mouse embryonic flibroblasts demonstrated increased PTEN biosensor BRET and this was associated with increased pAKT signalling ( Fig. 5f,g ). The findings above demonstrate that the biosensor can be used as readout for conformational change associated with PTEN activation status, following modulation of signalling pathways or interaction with PTEN-binding partners. 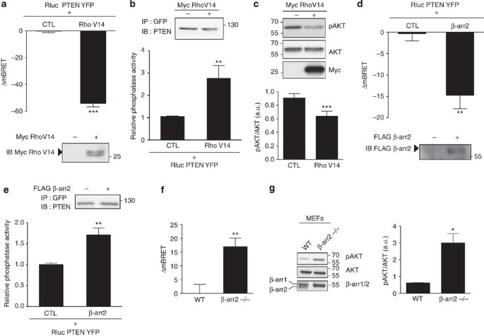Figure 5: Conformational changes of Rluc-PTEN-YFP induced by active RhoA and β-arr2 are associated with its activation status. (a) ΔmBRET values for Rluc-PTEN-YFP in HEK cells cotransfected with either empty vector or Myc-RhoV14. Graph represents means for five independent experiments±s.e.m. ***P<0.001,t-test. (b)In vitrolipid phosphatase activitiy of immunoprecipitated PTEN biosensor, using an anti-green fluorescent protein (GFP) antibody, from HEK293 cells transfected with Rluc-PTEN-YFP, or Rluc-PTEN-YFP and Myc-RhoV14. YFP vector control values were subtracted and samples normalized to PTEN alone. Data shown represents mean±s.e.m. of three independent experiments. **P<0.01,t-test. (c) Serum-starved HEK cells transfected with empty vector or Myc-RhoV14 were assessed for pAKT levels. Data shown represents mean±s.e.m. of six independent experiments. a.u., arbitrary units. ***P<0.001,t-test. (d) ΔmBRET values for Rluc-PTEN-YFP in HEK cells cotransfected with either empty vector or FLAG-β-arr2. Graph represents means for five independent experiments±s.e.m. **P<0.01,t-test. (e)In vitrolipid phosphatase activity of immunoprecipitated PTEN, using an anti-GFP antibody, from HEK293 cells transfected with Rluc-PTEN-YFP, or Rluc-PTEN-YFP and FLAG-β-arr2. YFP vector control values were subtracted and samples normalized to PTEN alone. Data shown represents mean±s.e.m. of three independent experiments. **P<0.01,t-test. (f) ΔmBRET values for Rluc-PTEN-YFP in WT or β-arr2−/− mouse embryonic flibroblasts (MEFs) transfected with Rluc-PTEN-YFP. Graph represents means for four independent experiments±s.e.m. **P<0.01,t-test. (g) WT and β-arr2−/− MEFs were assessed for pAKT levels. Data shown represents mean±s.e.m. of four independent experiments. a.u., arbitrary units. *P<0.05,t-test. BRET measurements in these experiments were performed on detached cells. Figure 5: Conformational changes of Rluc-PTEN-YFP induced by active RhoA and β-arr2 are associated with its activation status. ( a ) ΔmBRET values for Rluc-PTEN-YFP in HEK cells cotransfected with either empty vector or Myc-RhoV14. Graph represents means for five independent experiments±s.e.m. *** P <0.001, t -test. ( b ) In vitro lipid phosphatase activitiy of immunoprecipitated PTEN biosensor, using an anti-green fluorescent protein (GFP) antibody, from HEK293 cells transfected with Rluc-PTEN-YFP, or Rluc-PTEN-YFP and Myc-RhoV14. YFP vector control values were subtracted and samples normalized to PTEN alone. Data shown represents mean±s.e.m. of three independent experiments. ** P <0.01, t -test. ( c ) Serum-starved HEK cells transfected with empty vector or Myc-RhoV14 were assessed for pAKT levels. Data shown represents mean±s.e.m. of six independent experiments. a.u., arbitrary units. *** P <0.001, t -test. ( d ) ΔmBRET values for Rluc-PTEN-YFP in HEK cells cotransfected with either empty vector or FLAG-β-arr2. Graph represents means for five independent experiments±s.e.m. ** P <0.01, t -test. ( e ) In vitro lipid phosphatase activity of immunoprecipitated PTEN, using an anti-GFP antibody, from HEK293 cells transfected with Rluc-PTEN-YFP, or Rluc-PTEN-YFP and FLAG-β-arr2. YFP vector control values were subtracted and samples normalized to PTEN alone. Data shown represents mean±s.e.m. of three independent experiments. ** P <0.01, t -test. ( f ) ΔmBRET values for Rluc-PTEN-YFP in WT or β-arr2−/− mouse embryonic flibroblasts (MEFs) transfected with Rluc-PTEN-YFP. Graph represents means for four independent experiments±s.e.m. ** P <0.01, t -test. ( g ) WT and β-arr2−/− MEFs were assessed for pAKT levels. Data shown represents mean±s.e.m. of four independent experiments. a.u., arbitrary units. * P <0.05, t -test. BRET measurements in these experiments were performed on detached cells. Full size image Rluc-PTEN-YFP uncovers novel GPCR-mediated PTEN regulation Only a handful of receptors are currently known to physiologically regulate PTEN. One of these is the sphingosine 1-phosphate receptor 2 (S1PR2), which belongs to the GPCR family. The S1PR2 stimulates PTEN activity downstream of a RhoA-dependent pathway to inhibit cell migration [33] . Although the S1PR2 can stimulate PTEN activity in HEK cells, the related S1PR1 isoform was found to be without effect on PTEN activation [33] . We took advantage of these findings to test whether the lipid S1P acting at either the S1PR1 or S1PR2 expressed at equivalent levels ( Supplementary Fig. 3 ) could promote changes in PTEN conformation. HEK cells cotransfected with Rluc-PTEN-YFP and either S1PR1 or S1PR2 were incubated with S1P and BRET signals measured. Remarkably, whereas S1P (not vehicle alone) produced a change in BRET signal of Rluc-PTEN-YFP in S1P2R-expressing cells, S1P remained without effect in S1PR1-expressing cells ( Fig. 6a ). Similar BRET results were obtained in HeLa cells ( Fig. 6b ). Although the BRET experiments were performed with transfected receptors to bias signalling via the expressed receptor, we also pre-incubated untransfected HeLa cells, which endogenously express S1PR1 and S1PR2, with the specific S1PR2 antagonist and found that this led to increased AKT activation following incubation of cells with S1P ( Fig. 6c ). This is consistent with S1PR2-specific release of a PTEN-mediated brake on PI3K/AKT signalling in this cell model. 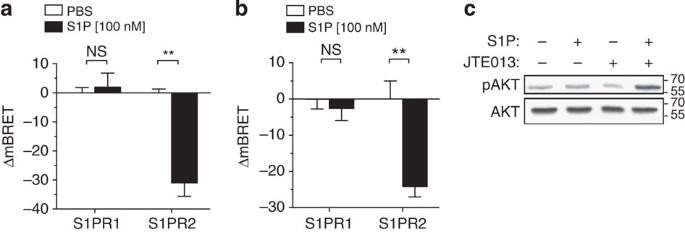Figure 6: S1PR2-induced PTEN conformational rearrangement monitored by real-time BRET. HEK (a) or HeLa cells (b) were cotransfected with Rluc-PTEN-YFP and S1PR1 or S1PR2, and treated with S1P (100 nM) or vehicle (PBS). Graphs represent ΔmBRET measurements att=5 min as mean±s.e.m. for four independent experiments. **P<0.01,t-test, n.s., not significant. (c) HeLa cells were preincubated with the S1PR2-specific antagonist JTE013 (1 μM) and then treated with S1P for 5 min. Cells were lysed and assessed for active AKT (pAKT) levels. BRET measurements in these experiments were performed on adherent cells. Figure 6: S1PR2-induced PTEN conformational rearrangement monitored by real-time BRET. HEK ( a ) or HeLa cells ( b ) were cotransfected with Rluc-PTEN-YFP and S1PR1 or S1PR2, and treated with S1P (100 nM) or vehicle (PBS). Graphs represent ΔmBRET measurements at t =5 min as mean±s.e.m. for four independent experiments. ** P <0.01, t -test, n.s., not significant. ( c ) HeLa cells were preincubated with the S1PR2-specific antagonist JTE013 (1 μM) and then treated with S1P for 5 min. Cells were lysed and assessed for active AKT (pAKT) levels. BRET measurements in these experiments were performed on adherent cells. Full size image We next used Rluc-PTEN-YFP as a screening tool in an attempt to uncover additional GPCRs capable of modulating PTEN function. As the S1PR2 activates PTEN via a RhoA-dependent pathway [33] , we tested several other GPCRs, known to stimulate RhoA-dependent signalling in HEK cells but that have not been reported so far to modulate PTEN activity in this system. The angiotensin type 1A receptor (AT1AR) has previously been shown to activate RhoA in HEK cells [34] , [35] , [36] . We first confirmed that the AT1AR can activate the Rho/ROCK pathway in HEK cells using an in vitro assay that measures ROCK activity. Following activation of the receptor by angiotensin II, cells were lysed, ROCK was immunoprecipitated and incubated with purified myosin phosphatase target subunit, as substrate, in the presence of ATP. Increased phosphorylated myosin phosphatase target subunit levels were observed following stimulation of the receptor, reflecting the activation of the RhoA/ROCK pathway ( Fig. 7a ). Cells were next cotransfected with the AT1AR and Rluc-PTEN-YFP, and incubated with angiotensin II. Ligand-induced conformational change of PTEN was illustrated by a significant decrease ( P <0.001, n =5, analysis of variance with Bonferroni post hoc test) in BRET at 5, 10 and 20 min incubation with angiotensin II compared with vehicle-treated cells ( Fig. 7b ). Raw Rluc and YFP emissions were not affected by treatment with angiotensin II ( Supplementary Fig. 4a,b ) confirming that the change in BRET was indeed due to conformational change. PTEN catalytic activity was found to increase over the same time frame using an in vitro phosphatase assay conducted in parallel ( Fig. 7c and Supplementary Table 1a ). Further evidence in favour of PTEN activation downstream of the AT1AR was also provided using a small interfering RNA (siRNA) approach to reduce PTEN levels. In control cells transfected with non-targeting siRNA, stimulation of the AT1AR by angiotensin II led to increased pAKT levels ( Fig. 7d ). Reduction of PTEN levels by siRNA led to increased basal pAKT levels, which were further increased on AT1AR activation ( Fig. 7d ). Taken together, the above results suggest a novel negative feedback loop on PI3K/AKT signalling and imply that PTEN activation can be triggered downstream of the AT1AR. 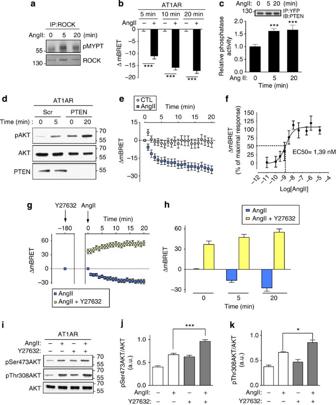Figure 7: AT1AR-induced PTEN activation monitored by real-time BRET. (a) ROCK activity was assessed, after AngII treatment, by immunoprecipitation of ROCK followed by incubation with its substrate, myosin phosphatase target subunit (MYPT). (b) HEK cells were cotransfected with Rluc-PTEN-YFP and AT1AR, and treated with AngII (100 nM). Graph represents the means±s.e.m. of three independent experiments. ***P<0.001,t-tests. (c) PTEN activity measuredin vitrofollowing AngII (100 nM) stimulation in HEK cells cotransfected with Rluc-PTEN-YFP and AT1 AR. Rluc-PTEN-YFP was immunoprecipitated using an anti-green fluorescent protein (GFP) antibody and incubated with water-soluble diC8-PIP3 (100 μM). YFP vector control values were subtracted and samples normalized to PTEN alone. Graph represents the means±s.e.m. of three independent experiments. ***P<0.001, analysis of variance with Bonferronipost hoctest. (d) HeLa cells were cotransfected with AT1AR and control or PTEN-targeting siRNA. Cells were left unstimulated or stimulated with AngII (100 nM) before being assessed for pAKT and PTEN levels. (e) Real-time analysis of ligand-induced conformational changes. HEK cells were cotransfected with Rluc-PTEN-YFP and AT1AR, and treated with AngII (100 nM). BRET readings were collected immediately after addition of agonist. Graph represents the means±s.e.m. of five independent experiments. (f) HEK cells were cotransfected with Rluc-PTEN-YFP and AT1AR, and treated with increasing concentrations of AngII for 10 min. Data were plotted using non-linear regression. Graph represents the means±s.e.m. of five independent experiments. (g) HEK cells were cotransfected with Rluc-PTEN-YFP and AT1AR, and pretreated with ROCK inhibitor Y27632 (10 μM) for 3 h before AngII stimulation. In the kinetic, cells are normalized to control cells at time 0. Data represent the means±s.e.m. of five independent experiments. (h) Histogram representation of data ingat 0, 5 and 20 min, showing ΔmBRET normalized to control cells att=0 min. (i) HeLa cells were transfected with AT1AR and pretreated with ROCK inhibitor Y27632 (10 μM) for 3 h before AngII stimulation. Cells were subsequently lysed and assessed for pAKT levels. Quantification of four independent experiments for phosphorylation of AKT at two sites is shown injandk. A.U., arbitrary units. Error bars are s.e.m. ***P<0.001, *P<0.05, analysis of variance with Bonferronipost hoctest. BRET measurements were performed on adherent cells. Figure 7: AT1AR-induced PTEN activation monitored by real-time BRET. ( a ) ROCK activity was assessed, after AngII treatment, by immunoprecipitation of ROCK followed by incubation with its substrate, myosin phosphatase target subunit (MYPT). ( b ) HEK cells were cotransfected with Rluc-PTEN-YFP and AT1AR, and treated with AngII (100 nM). Graph represents the means±s.e.m. of three independent experiments. *** P <0.001, t -tests. ( c ) PTEN activity measured in vitro following AngII (100 nM) stimulation in HEK cells cotransfected with Rluc-PTEN-YFP and AT1 AR. Rluc-PTEN-YFP was immunoprecipitated using an anti-green fluorescent protein (GFP) antibody and incubated with water-soluble diC8-PIP3 (100 μM). YFP vector control values were subtracted and samples normalized to PTEN alone. Graph represents the means±s.e.m. of three independent experiments. *** P <0.001, analysis of variance with Bonferroni post hoc test. ( d ) HeLa cells were cotransfected with AT1AR and control or PTEN-targeting siRNA. Cells were left unstimulated or stimulated with AngII (100 nM) before being assessed for pAKT and PTEN levels. ( e ) Real-time analysis of ligand-induced conformational changes. HEK cells were cotransfected with Rluc-PTEN-YFP and AT1AR, and treated with AngII (100 nM). BRET readings were collected immediately after addition of agonist. Graph represents the means±s.e.m. of five independent experiments. ( f ) HEK cells were cotransfected with Rluc-PTEN-YFP and AT1AR, and treated with increasing concentrations of AngII for 10 min. Data were plotted using non-linear regression. Graph represents the means±s.e.m. of five independent experiments. ( g ) HEK cells were cotransfected with Rluc-PTEN-YFP and AT1AR, and pretreated with ROCK inhibitor Y27632 (10 μM) for 3 h before AngII stimulation. In the kinetic, cells are normalized to control cells at time 0. Data represent the means±s.e.m. of five independent experiments. ( h ) Histogram representation of data in g at 0, 5 and 20 min, showing ΔmBRET normalized to control cells at t =0 min. ( i ) HeLa cells were transfected with AT1AR and pretreated with ROCK inhibitor Y27632 (10 μM) for 3 h before AngII stimulation. Cells were subsequently lysed and assessed for pAKT levels. Quantification of four independent experiments for phosphorylation of AKT at two sites is shown in j and k . A.U., arbitrary units. Error bars are s.e.m. *** P <0.001, * P <0.05, analysis of variance with Bonferroni post hoc test. BRET measurements were performed on adherent cells. Full size image BRET can monitor changes in energy transfer in real-time [27] . Next, we assessed the kinetics of changes in intramolecular BRET with Rluc-PTEN-YFP, following stimulation of the AT1AR in real-time by monitoring the same cell population and taking BRET measurements every minute. Using this approach, angiotensin II induced a time-dependent decrease in BRET over a 20-min time period, whereas no decrease in BRET was observed in control cells incubated with vehicle alone ( Fig. 7e ). A dose–response experiment was also performed ( Fig. 7f ) with varying angiotensin II concentrations at a fixed time point (10 min) and the obtained EC50 of 1.39 nM agrees well with data measuring EC50 values of angiotensin II on other downstream signalling events [37] . Pretreatment of cells with the ROCK inhibitor Y27632 enhanced the BRET signal above baseline levels (+37 mBRET) and abolished the time-dependent decrease in BRET following angiotensin II stimulation ( Fig. 7g,h ), demonstrating that activation of the biosensor occurs as a consequence of a cellular signalling cascade that regulates PTEN. In agreement with this, maximal AT1AR-induced pAKT levels at both Thr308 and Ser473 sites were higher following pretreatment of cells with Y27632 ( Fig. 7i,j ). We subsequently tested two other GPCRs, the thromboxane A2 receptor (TPαR) and the muscarinic M1 receptor (M1MR) known for their capacity to activate RhoA in HEK cells [38] , [39] . Following activation, both receptors produced significant shifts ( P <0.001, n =5) in BRET signal of Rluc-PTEN-YFP ( Fig. 8a,b ). Reduction of PTEN levels by siRNA led, in both cases, to higher pAKT levels following agonist stimulation, indicating that PTEN activity limits the PI3K/AKT pathway downstream of TPαR and M1MR signalling ( Fig. 8c,d ). Interestingly, in agreement with our findings here, TPαR was reported to activate PTEN in endothelial cell systems [40] . The above data provide proof of principle that receptor-mediated physiological regulation of PTEN can be detected using the PTEN biosensor. 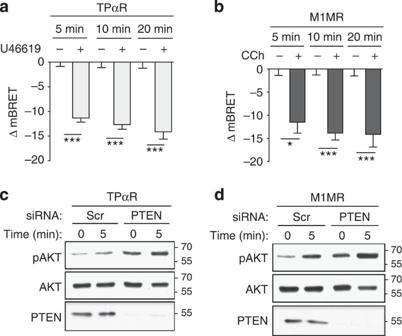Figure 8: TPαR and M1MR-induced PTEN activation monitored by real-time BRET. (a,b) HEK cells were cotransfected with Rluc-PTEN-YFP and TPαR or M1MR, and treated with thromboxane mimetic U46619 (1 μM) or Carbachol (CCh) (100 μM). Graphs represent the means±s.e.m. of three independent experiments. ***P<0.001, *P<0.05,t-tests. (c,d) HeLa cells were cotransfected with TPαR or M1MR, and control or PTEN-targeting siRNA. Cells were left unstimulated or stimulated with U46619 (1 μM) or Carbachol (CCh) (100 μM) before being lysed and assessed for pAKT and PTEN levels by western blotting. BRET measurements in these experiments were performed on adherent cells. Figure 8: TPαR and M1MR-induced PTEN activation monitored by real-time BRET. ( a , b ) HEK cells were cotransfected with Rluc-PTEN-YFP and TPαR or M1MR, and treated with thromboxane mimetic U46619 (1 μM) or Carbachol (CCh) (100 μM). Graphs represent the means±s.e.m. of three independent experiments. *** P <0.001, * P <0.05, t -tests. ( c , d ) HeLa cells were cotransfected with TPαR or M1MR, and control or PTEN-targeting siRNA. Cells were left unstimulated or stimulated with U46619 (1 μM) or Carbachol (CCh) (100 μM) before being lysed and assessed for pAKT and PTEN levels by western blotting. BRET measurements in these experiments were performed on adherent cells. Full size image Monitoring PTEN function on therapeutic agent treatment To determine whether therapeutic agents that impact on PTEN function can be monitored using this biosensor, we tested for the effect of trastuzumab, a rationally designed targeted treatment for certain breast cancer patients [41] . Trastuzumab is a humanized antibody targeting ERBB2 that displays therapeutic efficacy in certain patients with ERBB2-overexpressing breast tumours. PTEN has been reported to contribute to the antitumour activity of trastuzumab [42] , patients harbouring PTEN-deficient breast cancers showing significantly poorer responses to this antibody than those with normal PTEN. Acute trastuzumab treatment of breast cancer cell lines overexpressing endogenous ERBB2, results in increased membrane association and phosphatase activity of PTEN with consequent downregulation of pAKT levels [42] . We expressed Rluc-PTEN-YFP in SKBR3 breast cancer cells, which express high levels of endogenous ERBB2, and in MCF7 cells, which do not ( Fig. 9a ). Incubation of SKBR3 cells with trastuzumab resulted in decreased BRET signals, which was maximal at 20 min ( Fig. 9a ). The change in BRET signal coincided with increased PTEN activity ( Fig. 9b and Supplementary Table 1b ) and decreased cellular pAKT levels ( Fig. 9c ). Incubation of MCF-7 cells with trastuzumab did not result in any significant change in BRET compared with baseline values, suggesting that the effect of trastuzumab in SKBR3 cells does indeed pass through ERBB2 ( Fig. 9a ). To further confirm the specificity of the response obtained with the biosensor, we used MCF-7 cells stably transfected with either full-length ERBB2 or p95-ERBB2, an amino-terminally truncated receptor that is found in some tumours and that cannot bind to trastuzumab [43] . A 20-min incubation with trastuzumab caused a change in BRET signal in full-length ERBB2-expressing cells but no change was observed in the p95-ERBB2-expressing cells lacking the trastuzumab-binding extracellular domain ( Fig. 9d ). These data illustrate the specificity of the biosensor, showing that while trastuzumab acting through the full-length ERBB2 receptors impacts PTEN, the p95-ERBB2 receptor that is refractory to trastuzumab does not. 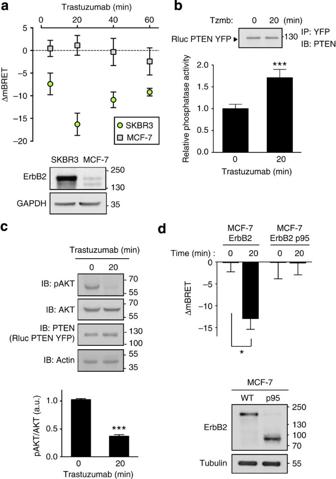Figure 9: Trastuzumab induces conformational changes that correlate with enhanced lipid phosphatase activity of PTEN. (a) BRET experiment in SKBR3 and MCF-7 cells transfected with Rluc-PTEN-YFP and treated with trastuzumab (2 μg ml−1) for the indicated times. Graph represents means±s.e.m. for four independent experiments. Lower panel shows representative western blotting using an anti-ErbB2 antibody on lysates of SKBR3 and MCF-7 cells. GAPDH was used as loading control. (b)In vitrophosphatase assay of immunoprecipitated Rluc-PTEN-YFP from transfected SKBR3 treated with Trastuzumab for 20 min (2 μg ml−1). YFP vector control values were subtracted and samples normalized to PTEN alone. Graph represents the mean±s.e.m. of three independent experiments ***P<0.001,t-test. (c) Levels of activated Akt (pAkt) assessed in SKBR3 cells. Cells were transfected with Rluc-PTEN-YFP and treated with Trastuzumab (2 μg ml−1). a.u., arbitrary units. Graph represents the mean±s.e.m. of four independent experiments *P<0.05,t-test. (d) MCF-7 cells stably transfected with ErbB2 or the truncated ErbB2 p95 variant were transiently transfected with Rluc-PTEN-YFP and treated with trastuzumab (2 μg ml−1) for the indicated times. Graph represents means±s.e.m. for four independent experiments, *P<0.05,t-test. Lower panel shows representative western blotting using an anti-ErbB2 antibody on lysates. Tubulin was used as loading control. BRET measurements in these experiments were performed on adherent cells. Figure 9: Trastuzumab induces conformational changes that correlate with enhanced lipid phosphatase activity of PTEN. ( a ) BRET experiment in SKBR3 and MCF-7 cells transfected with Rluc-PTEN-YFP and treated with trastuzumab (2 μg ml −1 ) for the indicated times. Graph represents means±s.e.m. for four independent experiments. Lower panel shows representative western blotting using an anti-ErbB2 antibody on lysates of SKBR3 and MCF-7 cells. GAPDH was used as loading control. ( b ) In vitro phosphatase assay of immunoprecipitated Rluc-PTEN-YFP from transfected SKBR3 treated with Trastuzumab for 20 min (2 μg ml −1 ). YFP vector control values were subtracted and samples normalized to PTEN alone. Graph represents the mean±s.e.m. of three independent experiments *** P <0.001, t -test. ( c ) Levels of activated Akt (pAkt) assessed in SKBR3 cells. Cells were transfected with Rluc-PTEN-YFP and treated with Trastuzumab (2 μg ml −1 ). a.u., arbitrary units. Graph represents the mean±s.e.m. of four independent experiments * P <0.05, t -test. ( d ) MCF-7 cells stably transfected with ErbB2 or the truncated ErbB2 p95 variant were transiently transfected with Rluc-PTEN-YFP and treated with trastuzumab (2 μg ml −1 ) for the indicated times. Graph represents means±s.e.m. for four independent experiments, * P <0.05, t -test. Lower panel shows representative western blotting using an anti-ErbB2 antibody on lysates. Tubulin was used as loading control. BRET measurements in these experiments were performed on adherent cells. Full size image Combined, the above data demonstrate that changes in BRET signal from the PTEN biosensor can reflect intramolecular conformational rearrangement that correlates with PTEN activation following physiological or therapeutic receptor engagement. The Rluc-PTEN-YFP biosensor described here can be used to rapidly detect conformational rearrangements of PTEN in intact cells and in real time, including those during its activation. Importantly, the biosensor retains PTEN catalytic activity and thus the capacity to downregulate the PI3K/AKT pathway, as well as displaying its expected cellular localization. A strong and stable intramolecular BRET was detected over a 100-fold range in expression, demonstrating the robustness of the biosensor. Moreover, BRET signals of Rluc-PTEN-YFP were detected at physiologically relevant levels of expression, following recomplementation of PTEN-null cells with the biosensor, to those that approximate endogenous expression in other PTEN-containing cells, highlighting its sensitivity. Receptors previously shown to be without effect on PTEN function did not produce changes in biosensor signal, demonstrating its specificity. We were also able to use Rluc-PTEN-YFP in a reporter role to uncover novel GPCR-mediated regulation of PTEN. Furthermore, activation-associated changes in Rluc-PTEN-YFP signal could be modulated pharmacologically with compounds targeting signalling pathways that impact PTEN function or by modifying therapeutic target receptor levels, as in the case of cell lines expressing different levels of ERBB2. However, as conformational changes detectable with the biosensor do not always necessarily reflect PTEN activation, for every new experimental setup BRET data need to be matched with additional tests, such as subcellular localization of PTEN or determination of active AKT levels. We used Rluc-PTEN-YFP in several different ways to investigate cellular and molecular mechanisms controlling the PTEN pathway. The biosensor was used in a structure–function mode to investigate whether mutation of amino acids implicated in the regulation of PTEN function results in conformational change in live cells. We demonstrated this by mutation of key amino acids in the C-terminal tail, known to be important for conformational rearrangement of PTEN, which also result in changes in its membrane targeting/cellular activity and found shifts in BRET signals of the biosensor, indicative of conformational change. Furthermore, we showed that pharmacological inhibition of CK2 caused changes in wild-type PTEN biosensor BRET signal that parallelled dephosphorylation of the regulatory C-terminal residues. This is of particular interest given that CK2 inhibition has been shown to restore PTEN-dependent signalling in cancer cell systems and has been suggested as a potential research avenue for T-ALL treatment [25] . Our data validate experimentally, in living cells, the proposed model of a PTEN switch between an open/active conformation targeted to the plasma membrane and a closed/less active cytoplasmic state [17] , [21] . The importance of PTEN membrane localization is highlighted by studies showing that certain cancer-associated mutations do not display reduced catalytic activity in vitro , but instead affect membrane localization [44] . The impaired plasma membrane binding of these mutants results in a PTEN-null phenotype in cells. The biosensor could, therefore, be used to probe the effects of other amino acids implicated in PTEN control, such as those that are the target of other post-translational modifications, in addition to assessing the effect of cancer-derived mutations on conformation. To provide an example of this, we investigated mutations that have previously been shown to ablate major mono-ubiquitination sites in PTEN. K13 in PTEN is mutated to glutamic acid (K13E) in spontaneous cancer [45] and K289 mutated to glutamic acid (K289E) is associated with Cowden syndrome [46] , [47] . These sites are found on unstructured regions of PTEN [14] ( Supplementary Fig. 5a,b ) and were both identified as major monoubiquitination sites that are important for nuclear import of PTEN [46] . Introduction of the K13E/K289E mutations in the Rluc-PTEN-YFP caused a change in BRET signal indicative of conformational change ( Supplementary Fig. 5 ). This indicates that in addition to reporting on phosphorylation-related changes in PTEN function, the BRET reporter can also be used to probe conformational changes associated with other post-translational modifications. The biosensor was also used to assess whether PTEN–protein partner interactions and/or important intracellular signalling proteins can induce PTEN conformational changes. As proof of concept, RhoA and β-arr2, known to activate PTEN [11] , [22] , both promoted changes in PTEN conformation in live cells. PTEN has a number of protein-binding partners that are required for its cellular functions and plasticity [1] , [48] , [49] , [50] , [51] . Previously characterized or candidate PTEN–protein partners that may form part of the PTEN interactome, as well as signalling proteins that may affect PTEN function, can therefore be rapidly assessed for their effect on PTEN conformation change by simple coexpression with Rluc-PTEN-YFP in live cells. It should be noted that a subset of PTEN partners that interact with PTEN through its C-terminal PDZ-binding sequence are probably not adapted to this approach due to the C-terminal fusion of YFP. The biosensor proved to be valuable in monitoring PTEN conformational change in real-time kinetic experiments in live cells, following incubation with therapeutic agents or physiological ligands that target cell surface receptors. Src is known to interact with ERBB2 and is therefore activated in ERBB2-overexpressing cancer cells [52] . PTEN function is inhibited by phosphorylation on tyrosine residues by Src family kinases [23] , [24] . The ERBB2-targeting antibody, trastuzumab, used in the treatment of certain breast cancers [41] , [42] induces PTEN membrane targeting and phosphatase activity by reducing PTEN tyrosine phosphorylation via Src inhibition [42] . We showed that trastuzumab caused a time-dependent change in Rluc-PTEN-YFP BRET that coincided with PTEN activation. The specificity of this signal was demonstrated by performing control experiments in cells that do not overexpress endogenous ERBB2, or in cells overexpressing a variant of the ERBB2 receptor, ERBB2-p95, which lacks the trastuzumab-binding extracellular domain [43] . We also probed the effect of several GPCRs for their effects on the biosensor. Whereas the lipid S1P was able to change the BRET signal of the biosensor through the S1PR2, it was without effect on the S1PR1 isoform, in agreement with previous finding that S1PR2, but not S1PR1, activates PTEN in HEK cells [33] . Using the same strategy, we were also able to identify three other GPCRs (AT1AR, TPαR and M1MR) that can activate PTEN. These experiments therefore provide proof of principle that the biosensor can be used to uncover additional cell surface receptors that influence PTEN function and provide a strategy for the identification of other potential physiological/therapeutic receptor targets. Finally, as the biosensor can be used as a rapid, direct and sensitive means to detecting activation of PTEN catalytic activity, it could therefore be used as readout for screening of small molecules that enhance or restore PTEN signal transduction. The identification of such agents would be potentially useful to manipulate PTEN signalling in a wide panel of human cancers. Plasmids and reagents Rluc-PTEN-YFP plasmid was generated by sequentially subcloning the coding sequence of Rluc in-frame at the N terminus and YFP at the C terminus of PTEN, yielding a Rluc-PTEN-YFP with flexible spacers of 18 amino acid between Rluc and PTEN, and 7 amino acid between PTEN and YFP. The sequential strategy allowed the generation of Rluc-PTEN and PTEN-YFP control vectors. Point mutations of PTEN in Rluc-PTEN-YFP were introduced by Quickchange (Stratagene) site-directed mutagenesis (PTEN-K13E/K289E) or by subcloning mutant PTEN (PTEN-A4) from previously characterized vectors. K13E was generated with the following primers: 5′-GTTAGCAGAAACGAAAGGAGATATCAAGAG-3′ (sense) and 5′-CTCTTGATATCTCCTTTCGTTTCTGCTAAC-3′ (anti-sense). K289E was generated with the following primers: 5′-GAAACCTCAGAAGAAGTAGAAAATGGA-3′ (sense) and 5′-TCCATTTTCTACTTCTTCTGAGGTTTC-3′ (antisense). Myc-PTEN, Myc-PTEN-A4, Myc-PTENΔtail (1–355) and Myc-RhoA-V14 constructs in the pRK5 vector were kind gifts of Alan Hall (MSKCC, New York). PTEN-tail (356–403)-YFP constructs were generated by amplifying the PTEN C-terminal tail by PCR and inserting the products into the pEYFP-N1 plasmid. All constructs were verified by sequencing (Institut Cochin Sequencing Facility). S1PR1, S1PR2 and TPαR were obtained from Missouri S&T complementary DNA resource centre. CK2 plasmid was obtained from David Litchfield (University of Western Ontario) via Addgene and has been described previously [53] . AT1AR and M1MR have been described previously [55] . The antibodies pAKT, total AKT, phospho PTEN (Ser380/Thr382/Thr383), PTEN (138G6), Myc (71D10), β-arr1/2 (D24H9), HA (C29F4) and GAPDH were from Cell Signalling; PTEN mAb clone 6H2.1 was from Millipore; green fluorescent protein and Myc (9E10) were from Roche; anti-c-erbB2 (clone e2-4001) was from Thermo Scientific; tubulin and actin were from Santa Cruz; and FLAG was from Sigma. All antibodies were used at 1/1,000 dilution for western blottings apart from anti-PTEN (138G6) and anti-β-arr1/2, which were used at 1/5,000 dilution. ROCK inhibitor Y27632, Carbachol and angiotensin II were from Sigma; U46619 and JTE013 were from Cayman Chemicals. Wheat-germ agglutinin–Texas Red conjugate was from Molecular Probes. Rho Kinase assay kit was from Cell Biolabs and Trastuzumab was kindly provided by Genentech. MCF-7 HER2 and p95 HER2 cells lines were a kind gift from Maurizio Scaltriti (Harvard Medical School). Cell culture and transfection All cell lines were obtained from the ATCC. HEK293T, HeLa and MCF-7 cells were cultured in DMEM medium supplemented with 10% fetal bovine serum (FBS) and penicillin/streptomycin. PC-3 cells were maintained in RPMI supplemented with 10% FBS and penicillin/streptomycin. SKBR3 cells were transfected with DMEM/F12 supplemented with 10% FBS and penicillin/streptomycin. HEK293T and HeLa cells were transfected using GeneJuice (Novagen), and SKBR3, MCF-7 and PC-3 cells were transfected with Fugene HD (Promega). Co-transfection of plasmids and siRNA in HeLa cells was performed using Dharmafect Duo. One microgram of plasmid and 100 nM final concentration of siRNA duplexes were used per well of a 12-well plate. PTEN phosphatase assay Phosphatase assays were performed as described previously [11] . Briefly, cells were transfected with either Rluc-PTEN-YFP or YFP vector and the indicated plasmids, lysates immunoprecipitated using an anti-PTEN antibody (Millipore) or an anti-green fluorescent protein antibody (Roche) and incubated 45 min at 37 °C with 100 μM water-soluble di-C8-PIP3 (Echelon Biosciences). Released phosphate was measured by optical density at 620 nm using Biomol green reagent (Enzo Life Sciences). YFP vector control values were subtracted and samples normalized to PTEN alone. Endogenous ROCK activity assay ROCK activity in cell lysates was measured using a kit from Cellbiolabs according to the manufacturer’s instructions. Immunoprecipitation and immunoblotting For co-immunoprecipitations of β-arr with Rluc-PTEN-YFP, cells were lysed in buffer containing 50 mM Hepes (pH 7.4), 250 mM NaCl, 2 mM EDTA, 0.5% NP-40, 10% glycerol supplemented with protease and phosphatase inhibitors (Roche) as used for previous β-arr interaction studies [21] , [54] , [55] . For co-immunoprecipitations of PTEN-tail fusions with PTEN-Δtail, HEK293T cells expressing relevant plasmids were lysed in buffer containing 10 mM Tris-HCl (pH 7.5), 140 mM NaCl, 5 mM EDTA and 0.1% Nonidet P-40 supplemented with protease and phosphatase inhibitors (Roche). For both immunoprecipitation protocols, lysates were cleared by centrifugation at 13,000 r.p.m. for 15 min at 4 °C. Supernatants were added to washed EZview Red Myc affinity beads (Sigma). Bound proteins were washed two to four times in lysis buffer and beads resuspended in Laemmli buffer. Immunoprecipitated proteins were subsequently detected by western blotting. Representative examples of uncropped western blottings are included in Supplementary Fig. 6 . Immunofluorescence Fluorescence microscopy was carried out using a Leica spinning-disk microscope with a × 63 oil immersion lens, equipped with a CoolSnap HQ2 charge-coupled device camera. Live images were acquired from HEK cells growing on 35 mm μ-dishes (Ibidi). HeLa cells were grown on glass coverslips for immunofluorescence and PC-3 cells were grown in Ibidi four-well chambers. BRET assays BRET assays were performed as described previously [27] , [28] , [56] . Briefly, 24 h post transfection, cells were detached with Hank’s balanced salt solution (Invitrogen) and distributed in white 96-well optiplates (Perkin Elmer). Coelenterazine h (Interchim) was added to a final concentration of 5 μM and incubated for 3 min at 25 °C. BRET readings were collected using a Multilabel Reader Mithras LB 940 (Berthold Technologies). Substrate and light emissions were detected at 480 nm (Rluc) and 540 nm (YFP) for 1 s. The BRET signal was calculated by ratio of the light emitted by YFP and the light emitted by Rluc (YFP/Rluc). The ratio values were corrected by substracting background BRET signals detected when Rluc-PTEN was expressed. mBRET values were calculated by multiplying these ratios by 1,000. For receptor stimulation assays with adherent cells, HEK cells were seeded in white 96-well culture plates (Perkin Elmer) 24 h before transfection. Cells were transfected with the indicated plasmids 24 h after seeding. Eight hours after transfection, cells were starved in DMEM without serum. Twenty four hours after transfection, medium was replaced by Hank’s balanced salt solution supplemented with 10 mM Hepes. Coelenterazine h was added to a final concentration of 5 μM and incubated for 3 min at 25 °C. The appropriate concentration of ligand was added after incubation and readings were collected immediately. Flow cytometry HeLa cells were re-suspended in PBS, 2% FBS fatty acid free and incubated with various concentration (0.1 nM–2 mM) of S1P-fluorescein-conjugated (Echelon) for 20 min or S1P-fluorescein-conjugated (Echelon) with 20 times more unconjugated S1P to measure the nonspecific binding. Data acquisition was performed on FACSCanto II (BD) flow cytometer and analysed with FlowJo software (Treestar). Specific mean fluorescence intensity was plotted against S1P concentration and B max was calculated from the scatchard plot generated on Graphpad Prism. Data analysis and statistics Where quantification is included for western blottings, signals were quantified by densitometric analysis using Image J. Data represented are the means±s.e.m. of a least three independent experiments. Statistical analysis was performed using GraphPad Prism software with either paired t -test or one-way analysis of variance with Bonferroni post hoc test. How to cite this article : Lima-Fernandes, E. et al. A biosensor to monitor dynamic regulation and function of tumour suppressor PTEN in living cells. Nat. Commun. 5:4431 doi: 10.1038/ncomms5431 (2014).